Abyssal undular vortices in the Eastern Mediterranean basin Abyssal temperature and velocity observations performed within the framework of the Neutrino Mediterranean Observatory, a project devoted to constructing a km 3 -scale underwater telescope for the detection of high-energy cosmic neutrinos, demonstrate cross-fertilization between subnuclear physics and experimental oceanography. Here we use data collected south of Sicily in the Ionian abyssal plain of the Eastern Mediterranean (EM) basin to show for the first time that abyssal vortices exist in the EM, at depths exceeding 2,500 m. The eddies consist of chains of near-inertially pulsating mesoscale cyclones/anticyclones. They are embedded in an abyssal current flowing towards North-Northwest. The paucity of existing data does not allow for an unambiguous determination of the vortex origin. A local generation mechanism seems probable, but a remote genesis cannot be excluded a priori . The presence of such eddies adds further complexity to the discussion of structure and evolution of water masses in the EM. Searching for a site suitable for the implementation of a neutrino detector, within the Neutrino Mediterranean Observatory (NEMO) project [1] , [2] , [3] , a long-term mooring was established to monitor oceanic abyssal currents in the Eastern Mediterranean (EM) basin at the KM4 site ( Fig. 1a ). Ocean dynamics possess 'elementary particles', often formed by closed circulations within distinct water masses that can propagate for long distances with small dissipation. They are considered to have an important role in the larger-scale oceanic circulation and variability [4] . 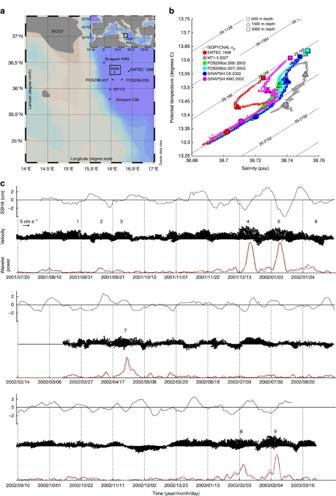Figure 1: Local thermohaline properties and observed currents in the study area. (a) Map of the Ionian basin in the approaches to the KM4 site, indicating the location of the conductivity–temperature–depth (CTD) stations from EMTEC cruise (April 1999), SINAPSI 4 cruise (April 2002), POSEIDON cruise 298 (May 2003) and M71/3 cruise (January 2007). (b) Potential temperature (θ)–salinity (S) diagram of CTD stations at the KM4 region between 1999 and 2007 from EMTEC, SINAPSI 4, POSEIDON 298 and M71/3 cruises. Squares indicate data at 800 m depth, upward-pointing triangles indicate data at 1,500 m depth and circles indicate data at 3,000 m depth. The isolines refer to the potential densityσ0. (c) Evolution of SSH anomalies at KM4 (SSHA, top), upper-level measured velocities during the whole 2002–2003 campaign at KM4 (stick arrows, middle) and wavelet power of associated meridional (black line) and zonal (red) velocity components around the inertial frequency band (non-dimensional, bottom). Numbers identify major episodes of enhanced mesoscale vortical activity. Figure 1: Local thermohaline properties and observed currents in the study area. ( a ) Map of the Ionian basin in the approaches to the KM4 site, indicating the location of the conductivity–temperature–depth (CTD) stations from EMTEC cruise (April 1999), SINAPSI 4 cruise (April 2002), POSEIDON cruise 298 (May 2003) and M71/3 cruise (January 2007). ( b ) Potential temperature ( θ )–salinity ( S ) diagram of CTD stations at the KM4 region between 1999 and 2007 from EMTEC, SINAPSI 4, POSEIDON 298 and M71/3 cruises. Squares indicate data at 800 m depth, upward-pointing triangles indicate data at 1,500 m depth and circles indicate data at 3,000 m depth. The isolines refer to the potential density σ 0 . ( c ) Evolution of SSH anomalies at KM4 (SSHA, top), upper-level measured velocities during the whole 2002–2003 campaign at KM4 (stick arrows, middle) and wavelet power of associated meridional (black line) and zonal (red) velocity components around the inertial frequency band (non-dimensional, bottom). Numbers identify major episodes of enhanced mesoscale vortical activity. Full size image During the EM Transient (EMT), a major climate shift that occurred at the end of the eighties and culminated in the nineties, relatively warm and salty abyssal waters of Aegean origin replaced colder and fresher Adriatic deep water (AdDW) in the bottom layers of the Ionian basin [5] , [6] . As a consequence, newly formed AdDW no longer possessed the density required to sustain its descent towards the Ionian abyss as a vein of bottom-arrested current as before the EMT. Instead, it had to intrude above waters of Aegean origin in the abyss of the northern and/or central Ionian basin [5] . This gave birth to profound transformations in the dynamics of AdDW and deep Aegean waters. Note that bottom-arrested currents, when they leave the ocean floor, transform themselves into intermediate currents and accordingly develop new dynamical features. Particularly, they can disintegrate into vortex chains, which can be advected by a background current [7] , [8] , [9] , [10] , [11] . Also as a consequence of such a complexity, in the Ionian basin, deep waters can differ considerably in their characteristics, dynamics and routes, which are partly determined by the underlying bathymetry [5] . Note also that the beginning of the new millennium can be considered as a period of large variability for water mass formation and stratification in the EM [5] , [6] , [12] , [13] , [14] , [15] , [16] . Variability inherent in the hydrodynamics of sea overflows, which can be baroclinically unstable [17] , adds complexity to this scenario. Numerical simulations confirm the existence of such a variability [17] , [18] , which is found also in the EM [19] . However, the capability of phenomena emerging from such complexity to preserve their coherence in the Ionian deep layers has yet to be demonstrated. Using the KM4 measurements, we show for the first time that abyssal vortex chains exist in the EM at depths exceeding 2,500 m. They consist of chains of undular mesoscale cyclones/anticyclones embedded in an abyssal current. An unambiguous determination of their origin is not allowed by the paucity of the existing data, therefore we discuss different hypotheses: a local generation mechanism seems probable, but a remote genesis cannot be excluded a priori . General properties of observed current metre data at KM4 Current metre data (at 2,700 m and 3,050 m depths) describing the abyssal circulation in the approaches to the KM4 site, a ∼ 3,350-m deep flat plain about 130 km south-east of the southern tip of Sicily ( Fig. 1a ), indicate the presence of a prevailing current towards NNW at ∼ 1.9 cm s −1 ( Fig. 1c ). The presence of such a background abyssal current in the region is consistent with previous studies [5] , [6] , [13] , [14] , [20] suggesting that, as a part of the EMT, waters of Aegean origin replaced waters of Adriatic origin in the abyssal plain of the Ionian basin (see Fig. 1b ). Note that, in addition to this shift, which could belong to a part of a larger mode of variability of the EM [21] , a substantial mesoscale, interseasonal and interannual variability exists in EM water masses formation and circulation [5] , [6] , [13] , [14] , [20] , [22] . Evidence of such a replacement is shown in the θ- S diagrams of Fig. 1b . The local deep waters, whose vertical structure suggests that between 1999 and 2003 its largest variability took place in an intermediate layer around 1,500 m depth, became warmer and saltier after 2003. Note that the thermohaline properties of the bottom layer did not show a large variability between 1999 and 2003. At the KM4 station, data show that deep currents superimposed on the average flow possess an undular character. They are characterized by quasi-inertial, tidal and mesoscale signals, whose major episodes are numbered in Fig. 1c . At both depths, measured in situ temperatures ( T ) show a rather constant background value ( ∼ 13.87 °C at the upper depth and ∼ 13.84 °C at the bottom depth, see Fig. 2c ) with superimposed temporally variable O (0.05 °C) cold pulses. 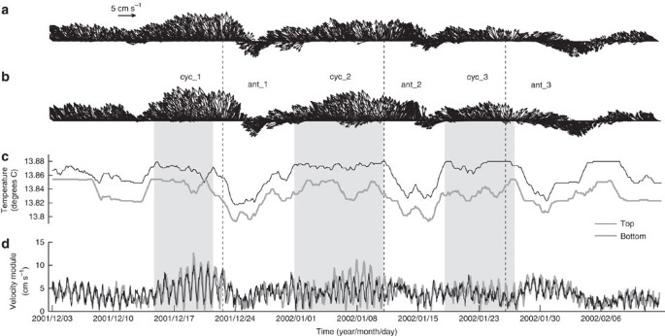Figure 2: Evidence of the passage of an undular vortex chain. Temporal evolution of top (a) and bottom (b) velocities,in situtemperatures (c) and velocity modules (d) measured at the KM4 site around the passage of vortical events nos. 4–6 inFig. 1c. The grey shading indicates periods when temperature is high and fairly constant; the dashed vertical lines indicate periods when the zonal velocity components evolve from preferentially westward to preferentially eastward. Cyclones (cyc) and anticyclones (ant) are numbered progressively. Figure 2: Evidence of the passage of an undular vortex chain. Temporal evolution of top ( a ) and bottom ( b ) velocities, in situ temperatures ( c ) and velocity modules ( d ) measured at the KM4 site around the passage of vortical events nos. 4–6 in Fig. 1c . The grey shading indicates periods when temperature is high and fairly constant; the dashed vertical lines indicate periods when the zonal velocity components evolve from preferentially westward to preferentially eastward. Cyclones (cyc) and anticyclones (ant) are numbered progressively. Full size image Evidence of the passage of mesoscale vortex chains at KM4 The most striking feature characterizing our time series is the occurrence of a chain of abyssal mesoscale vortices. The velocity field observed at the upper depth throughout the sampling period ( Fig. 1c ) evidences at least nine episodes of enhanced mesoscale undular vortical activity. Within each of these episodes, the velocity field seems to be composed of two distinct patterns. The first one consists of a mostly clockwise rotation, progressively intensifying in amplitude, followed by a progressive attenuation, resembling a fan shape (see Figs 1c and 2a,b ). The second one consists of an abrupt, full-circle clockwise rotation of the velocity field producing a sudden, temporarily southward orientation of the velocity vectors. Such composite basic patterns can either occur in isolation, as in the case of episode no. 7, or as a pair and even multiple composite events, as in the case of episode nos. 1–3 and 4–6 (see also Fig. 2 and the corresponding discussion below). The time needed for such composite patterns to be accomplished typically ranges from a few days to about two weeks. Intriguingly, these events tend to be associated to major departures of the measured T from its background average value. Particularly during a typical event entailing the two basic velocity pattern types in succession (that is, the fan structure and the full-circle rotation), T tends to stay fairly constant until the velocity field is directed northward and it decreases thereafter, remaining below-average until the velocity field entails a southward component ( Fig. 2a–c ). Details characterizing velocity and temperature anomaly evolutions, as measured at the two depths, further unveil valuable information about the nature and origin of such fluctuations. In general, the fluctuations extend upon the two depths, indicating that the anomalies correspond to coherent features spanning over several hundreds of metres in the vertical. Under the reasonable assumption that such anomalies are features advected by the background flow, their horizontal dimensions can be estimated to be O(10 km). Visual inspection of individual fluctuation patterns indicates that, in some cases, their beginning and ending times are not completely synchronous at the two depths (see, for example, the temperature evolutions in Fig. 2c ). Instead, they tend to be separated by lags spanning from several hours up to about 1 day. Often, when upper-depth signals anticipate lower-depth signals at the beginning of the fluctuation, they follow at the ending of the fluctuation. Furthermore, during such fluctuations, the temporal rate of change of temperature signals often differs at the two depths. This suggests that the spatial structures of the observed anomalies, at least during some of the recorded episodes, are consistent with those of lens-like vortices, preferentially centred above the average current metre depth. During these fluctuations, more energetic quasi-inertial peaks with respect to the undisturbed flow emerge ( Figs 1c and 2d ), which unveil the undular character of the vortices. The observed fields trace the passage of abyssal undular mesoscale vortices. We exclude that, in general, these features extend to the near-surface, as sea surface height (SSH) variability in the area (see Fig. 1c ) does not show a robust connection with the passage of the eddies. Some degree of correlation can be seen between observed SSH, bottom velocities and quasi-inertial energy distribution for episodes no. 4, no. 5 and no. 6 ( Fig. 1c ). However, as the observed signals are out of phase and SSH amplitudes are fairly small, we cannot confidently associate the observed surface anomalies to the abyssal eddies. The observed dynamics can be tentatively explained assuming the presence of trains of alternating cyclones/anticyclones, advected by a ∼ 1.9 cm s −1 background flow directed towards NNW, whose centres pass west of the monitoring site ( Fig. 3a ). The azimuthal velocity profiles of both cyclones and anticyclones are almost linear functions of the vortex radii in a core region and rapidly decay in an outer region ( Fig. 3b ). Notably, anticyclonic mesoscale vortical features characterized by similar radial structures of their tangential velocities describing internal undular oceanic vortices have been recently discovered as robust solutions of the non-stationary, nonlinear shallow-water equations on an f -plane [23] , [24] , [25] , [26] and also demonstrated as being persistent features of both oceanic and laboratory flow fields [27] , [28] . Remarkably, they are all characterized by the presence of (quasi) inertial pulsations, as those observed here to be significantly enhanced during vortical activity ( Fig. 1c ). The cores of the anticyclones we selected to mimic the observations are colder than surrounding waters ( Fig. 3b ). Intriguingly, similar temperature drops associated with mesoscale vortical activity were recently detected in the EM [19] . In the world ocean, lens-like mesoscale eddies are known to be able to transport temperature and salinity anomalies for long distances [4] . Here, as a mere conjecture, this kind of propagation would be consistent with injections of fresher, less-salty waters in the Ionian abyss, with its possibly associated physical and biogeochemical anomalies. 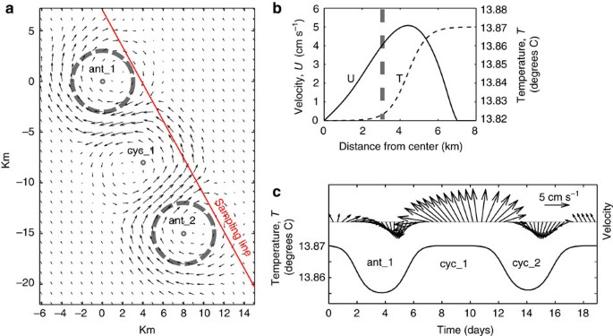Figure 3: Interpretation of measured velocity and temperature fields. (a) Velocity pattern associated with the passage of an anticyclone/cyclone/anticyclone train transported by a background flow of 1.9 cm s−1directed towards NNW. The red line indicates the sampling line. (b) Tangential velocity (U) and temperature (T, only for anticyclones) profiles characterizing the vortices. The vertical dashed line indicates the core of anticyclones (also shown in panela). (c) Temporal evolution of velocity and temperature as measured along the sampling line, mimicking the passage of the train of vortices to a fixed sampling site. Figure 3: Interpretation of measured velocity and temperature fields. ( a ) Velocity pattern associated with the passage of an anticyclone/cyclone/anticyclone train transported by a background flow of 1.9 cm s −1 directed towards NNW. The red line indicates the sampling line. ( b ) Tangential velocity ( U ) and temperature ( T , only for anticyclones) profiles characterizing the vortices. The vertical dashed line indicates the core of anticyclones (also shown in panel a ). ( c ) Temporal evolution of velocity and temperature as measured along the sampling line, mimicking the passage of the train of vortices to a fixed sampling site. Full size image The passage of an anticyclone/cyclone/anticyclone train transported by a background flow like that illustrated in Fig. 3a produces the velocity and temperature fields shown in Fig. 3c . The patterns bear a strong similarity with those illustrated in Fig. 2a–c , which are associated to the passage of antno.2/cycno.2/antno.3. In fact, the mimicked evolution entails an initial temporary shift of velocities towards south, linked to the passage of the first anticyclone, followed by a northward fan-shaped velocity structure, linked to the passage of the cyclone, and a second shift of velocities towards south linked to the passage of the second anticyclone. Remarkably, the mimicked temperature evolution closely traces the observed cooling phases linked to the passage of anticyclones: the onset of cold anomalies preludes to southward velocity inversions. Table 1 summarizes characteristics of the observed vortices [29] . Rossby number estimates span from ∼ 0.1 to ∼ 0.2, and they are larger for anticyclones, which is consistent with previous analyses of interior mesoscale vortices [29] . The presence of such eddies in the abyssal layers of the Ionian basin adds further complexity to the discussion of structure and evolution of water masses in the EM. Table 1 Characteristics of eddies illustrated in Fig. 2 evaluated from data collected on the KM4 top mooring. Full size table We note that Manca et al . [15] , [20] observed the arrival of deep water of Adriatic origin at the base of the Sicily escarpment during 1991 that was possibly able to produce some reversals in the main bottom flow, which, at the time, was dominated by an anticyclonic motion. However, these authors also pointed out that during 1999 the region was still occupied by waters of Aegean origin, as confirmed by other studies [14] , [30] . Figure 1b , on the other hand, does not show significant changes in the thermohaline properties of the bottom layer between 1999 and 2003. Owing to the paucity of the data, we are not able to unambiguously identify origin and generation mechanisms for the observed phenomena. A local recirculation, which could be favoured by the local bathymetry, characterized by the presence of a prominent, almost zonally oriented abyssal ridge in the region, seems probable. However, a more remote origin cannot be excluded a priori . If demonstrated, it would envisage the existence, in the Ionian basin, of deep water mass transport mechanisms beyond those already known to exist in conjunction with near-bottom current dynamics. Our investigation shows that efforts in very different disciplines, like subatomic physics and experimental oceanography, can be successful in producing new knowledge. In this case, the search for elusive elementary particles enabled the discovery of abyssal 'elementary' undular vortices in the EM. Dataset Current metre data were collected between July 2001 and March 2003 at 2,700 and 3,050 m depth at the KM4 site (36°19′N; 16°05′E). Current metres are Aanderaa RCM 11 characterized by a resolution of ∼ 0.05 °C for temperature, T , 0.3 cm s −1 for flow velocity and 0.35° for flow direction. A quality check was performed, specifically for removing spikes and instrumental failures. Owing to calibration problems affecting their accuracy, salinity data are not considered in this study. Conductivity–temperature–depth data used in this work refer to profiles conducted in the proximity of the KM4 station between 1999 and 2007. Specifically, they were acquired during EMTEC cruises (April–May 1999, station INT), SINAPSI-4 cruise (March–April 2002, stations C06 and KM3), Poseidon Cruise 298 (May 2003, stations 207 and 208) and Meteor Cruise M71-3(January/February 2007, station 103). The altimetre data used for this analysis are obtained from the AVISO (Archiving, Validation and Interpretation of Satellite Oceanographic data) Jason-2 Interim Geophysical Data Record products [31] . The Absolute Dynamic Topography data are obtained by referencing 46 measured SSHs with respect to a synthetic estimate of the geoid [32] . Plotted data were pre-processed using a 21-day moving window high-pass filter. Data analysis techniques To analyse quasi-inertial oscillations, the wavelet power spectra of the u and v components of measured velocity data were computed using the matlab wavelet toolbox available at the University of Colorado website: http://paos.colorado.edu/research/wavelets/software.html . The mother wavelet function adopted is the Morlet with non-dimensional frequency ω 0 =6. The considered band around the inertial frequency includes periodicities ranging from 19.65 to 20.34 h. The passage of a train of cyclones/anticyclones was mimicked by inspecting the values of a two-dimensional velocity and temperature fields along a sampling line. The velocity and temperature fields consist of a uniform background (13.87 °C for temperature, [ V , α ]=[1.9 cm s −1 , 2π/3] for velocity), with superimposed temperature and velocity anomalies associated with the presence of an anticyclone/cyclone/anticyclone train. The lines connecting the centres of the eddies and the sampling line were imposed to be parallel to the background velocity. The horizontal size of both cyclones and anticyclones is 7 km, with imposed peaking tangential velocity of O(5 cm s −1 ) at ∼ 4.5 km from the centre. Anticyclone cores, within 2 km from the centre, are associated to a 0.05 °C temperature drop. Eddy characteristics in Table 1 were estimated based on geometrical characteristics [29] . A stationary background flow of 1.9 cm s −1 strength and 2π/3 direction (that is, NNW) was assumed. To eliminate the effect of inertial fluctuations, daily average data were used for the estimation. How to cite this article: Rubino, A. et al . Abyssal undular vortices in the Eastern Mediterranean basin. Nat. Commun. 3:834 doi: 10.1038/ncomms1836 (2012).